Seismic insights into Earth’s core 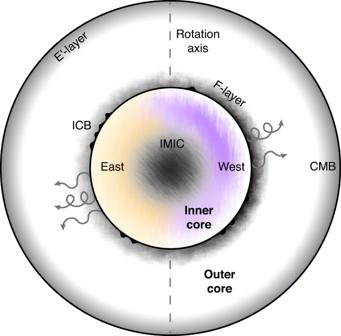Fig. 1: Stylised illustration of structures and processes in Earth’s core. The outer core radius is 3480 km, the inner core radius is 1220 km (to the nearest 10 km)3. Features denoted include: outer core stratification (the E’ and F- layers); inner core boundary topography and asymmetry of the F-layer; inner core hemispheres, anisotropy, and regional variation; and innermost inner core, distinctly different from the rest of the inner core. Arrows indicate the release of light elements upon inner core growth, colours and textures in the inner core signify the strength and nature of anisotropy, and shading in the outer core represents seismic velocity anomalies. Seismology’s limited observational resolution results from geographical constraints on the geometrical sampling of core-sensitive seismic waves and difficulties in isolating these small amplitude signals from noise [2] . New discoveries have employed both ever-increasing numbers of seismic stations and novel observational methods [6] , [7] . These techniques deliver information beyond traditional seismic methodologies, which primarily employ the arrival times and amplitudes of direct seismic waves [1] , [2] , [3] or information about whole-Earth vibrational frequencies [4] . A significant recent development introduced the concept of the global coda-correlation wavefield [6] , [8] , [9] , [10] , [11] . Its realisation, a correlogram, is constructed by cross-correlating and stacking late hours of seismic records following large earthquakes. The long-lasting global reverberations dramatically improve spatial coverage, and the method boosts the amplitude of weak signals, manifesting as cross-correlation peaks in correlograms [6] . They have proved ideal for new observations of the core structure, including measurements of inner core shear properties [6] , [8] , anisotropy of the IMIC [9] , [10] , and stratification of the outer core [11] . Another emerging approach uses transdimensional statistical tomography to produce 3D models of the core’s seismic properties, accompanied by uncertainty, simultaneously mapping quasi-hemispherical asymmetry, anisotropy, and regional-scale features [7] , [12] . Tomographic inversions for inner core structures are not new, but remain more challenging and less well-developed than mantle tomography. The most up-to-date inner core models contain large uncertainties, uneven spatial parameterisation, and theoretical errors from ambiguity in mantle structure [13] , so limitations on the resultant interpretations must be acknowledged [12] . We highlight here seismic structures emerging into focus within contemporary observational models, which provoke ongoing dynamical and compositional interpretations. Notable topics currently attracting discourse are inner core shear properties [3] , [6] , [8] , the IMIC [9] , [10] , [12] , [13] , and boundary layers [4] , [11] , [14] , [15] , [16] , [17] , yet inconsistencies remain in their reported properties. Inner core shear properties Seismic observations confirmed the inner core as solid in the 1970s, some 30 years after mineral physics arguments proposed its solidity [1] , [2] . The elusiveness of inner core shear waves has restricted their ability to constrain its shear properties [3] . Recent observations of shear waves in the coda-correlation wavefield have provided improved estimates of inner core shear velocity, anisotropy, and attenuation [6] , [8] , proposing lower velocity and, perhaps, stronger attenuation than previous values. Updated constraints on shear velocity anisotropy near the core’s centre find the direction of the highest wavespeeds oblique to Earth’s rotation axis, in contrast to compressional velocity anisotropy [8] . Observed shear properties of the inner core represent critical constraints for mineral physics experiments and calculations. Low shear velocity indicates softening of the inner core [5] , and the orientation of anisotropy helps ascertain candidate mineral phases of iron [1] , [2] , [3] . Improved geographical seismic coverage is needed for ongoing refinements to these measurements, including mapping radial and regional variations, fully calculating attenuation properties, and establishing the link to compressional velocity properties [6] , [8] . Innermost inner core (IMIC) Until recently, the IMIC was considered a possible artefact [1] , but current work is iterating towards a consensus for its properties. A few hundred kilometres in radius, the IMIC is characterised by different anisotropy from the bulk of the inner core, with a gradual transition between the two regions. Specifically, the IMIC has stronger velocity anisotropy, and a different direction of slowest wavespeed [9] , [10] , [13] . Although it has been proposed that the IMIC displays hemispherical asymmetry [1] , recent work argues that it may instead be shifted off-centre [12] , [13] . However, these two analyses define the IMIC with different criteria, using the polar-equatorial difference in wavespeed [13] versus the direction of slowest wavespeed [12] , and subsequently reach opposing conclusions for its position. Dynamically, the IMIC may mark a gradual transition in the growth processes of the inner core, observed as a change in the crystalline structure of iron [3] , [10] ; the relic of two-stage formation, also detected in paleomagnetic data [18] ; or the onset or cessation of external mechanisms creating texturing [13] . We anticipate ongoing improvements to the current IMIC models will provide the underpinning measurements to orient the next generation of core evolution models. Inner core boundary (ICB) We have considerably more data from the uppermost inner core than for deeper layers due to greater volumetric coverage and comparatively straightforward techniques to isolate the relevant signals [1] , [2] . The upper inner core demonstrates a distinct east-west dichotomy in its seismic velocity, the quasi-western hemisphere being slower for compressional waves by about 1%. Anisotropy is negligible in the outermost layers [1] , [2] , [3] , but increases considerably ~50 km beneath the ICB. It is thought to be confined to the western hemisphere [12] , although the current spatial coverage is far from complete. The ICB itself sustains localised topography of a few kilometres [2] , [14] . As the locus of inner core growth, the ICB region provides insight into current dynamical processes of the inner core and its interaction with the outer core [1] , [2] , [3] , [4] . Its features are ascribed to various dynamical mechanisms recorded in the inner core structure as it freezes [3] . For example, asymmetric heat flow could generate hemispherical differences in the inner core, with localised enhanced flux creating dynamical topography on the ICB and compositional heterogeneity in the F-layer [1] , [2] , [3] , [4] , [14] . Temporal variation of ICB topography and the uppermost IC may also arise from the differential rotation of the inner core with respect to the mantle [19] , [20] . This is difficult to detect seismically, hence there is currently no consensus on rotation and/or oscillation rate [1] , [2] , [3] , [14] , [19] , [20] . Outer core layering Layering may exist at both boundaries of the outer core. The ~100 km thick F-layer at its base exhibits a decreasing seismic velocity gradient [4] , [11] , and lateral variability [15] . In the uppermost outer core, the E’-layer displays a lower velocity anomaly relative to the well-mixed bulk of the outer core [3] , [4] , [11] , although studies disagree on its thickness [16] , [17] . Fluctuations in geomagnetic field strength and length-of-day measurements support the presence of stratification in the outermost outer core [21] . These data further indicate additional small-amplitude lateral variations in temperature and composition, but which are seismically undetectable [3] . Linking seismic models of the E’-layer to specific compositions is also not straightforward [5] . The existence of the F-layer is attributed to inner core growth mechanisms causing chemical stratification; for example, a partially-frozen slush snowing onto the ICB [3] . Localised melting or freezing of the ICB could create regional enrichment of iron or light elements. There are multiple options for generating a compositionally stratified E’-layer: remnants of core formation, interaction at the CMB, or light elements released upon inner core growth [3] . At the CMB, heat is extracted unevenly by the silicate mantle; seismic investigations of this dynamically important interface are an active research area [22] . As we face an unprecedented expansion of data sensitive to the deep Earth, seismic studies of the core are at a pivotal stage. We anticipate that the recent discoveries discussed here will precipitate further advancements in knowledge of core structures and dynamics. Potential near-future targets for core seismology include inner core shear wave attenuation, anisotropy, and tomography, high-resolution observations of boundary and transition layers, and improved tracking of temporal changes. Performing many of these analyses will be challenging, with several likely beyond the scope of present seismic detection techniques. Continual improvements in observational infrastructure and methodologies will therefore remain integral to the development of our understanding of the core. Coda-correlation [6] and machine learning algorithms [23] are emerging as valuable tools in studies of Earth’s inner layers, for seismic measurements, and their integration with outputs from other disciplines [24] . We anticipate that such data driven approaches will become prevalent for investigations into the core in coming years. Overall, interdisciplinary and multidisciplinary collaborations will be essential as we move forward in our attempts to understand Earth’s enigmatic core.